Separation of neutral and charge modes in one-dimensional chiral edge channels Coulomb interactions have a major role in one-dimensional electronic transport. They modify the nature of the elementary excitations from Landau quasiparticles in higher dimensions to collective excitations in one dimension. Here we report the direct observation of the collective neutral and charge modes of the two chiral co-propagating edge channels of opposite spins of the quantum Hall effect at filling factor 2. Generating a charge density wave at frequency f in the outer channel, we measure the current induced by inter-channel Coulomb interaction in the inner channel after a 3-μm propagation length. Varying the driving frequency from 0.7 to 11 GHz, we observe damped oscillations in the induced current that result from the phase shift between the fast charge and slow neutral eigenmodes. We measure the dispersion relation and dissipation of the neutral mode from which we deduce quantitative information on the interaction range and parameters. Most studies of collective excitations in one-dimensional (1D) systems performed so far have focused on non-chiral quantum wires [1] , [2] , [3] . In these systems, the collective excitations carrying the charge and the spin propagate at different velocities, leading to the separation of the charge and spin degrees of freedom. This spin-charge separation has been probed by measuring the tunnelling spectroscopy of individual electrons between a pair of 1D wires [1] , or alternatively, between a wire and a two-dimensional (2D) electron gas [3] . However, a direct observation of the collective modes is experimentally challenging as the relevant energy scales are too high for usual low-frequency measurements. The edge channels of the quantum Hall effect provide another implementation of 1D transport, where propagation is chiral and ballistic over large distances. These specificities have inspired several experiments that aim at reproducing, in solid state, optical setups where light beams are replaced by electron beams [4] , [5] , [6] , [7] . One major difference between electrons and photons comes from interaction effects, which are amplified in the 1D geometry and should enrich electron optics compared with its photonic counterpart. Of particular interest is the case of filling factor 2 where transport along the sample edge occurs through two co-propagating edge channels of opposite spins. Because of Coulomb interaction, the two edge states are coupled, and new propagating eigenmodes, with different velocities, appear [8] , [9] , [10] , [11] , [12] , similarly to the physics arising in 1D wires. Consequently, considering edge channels with the same propagation characteristics (but different spins), and denoting as the current components in edge channels 1 and 2 at position x and time t , a current ( i 1 , 0) in channel 1 decomposes in the symmetric fast charge mode and the antisymmetric slow neutral mode (also called dipolar mode). As these two modes propagate at different velocities, the current initially injected in channel 1 separates into the charge and the neutral modes of the two coupled edges. This mechanism is at the heart of the decoherence [9] , [10] , [13] and relaxation [14] , [15] , [16] , [12] of electronic excitations propagating in these systems. As such, it has been probed through Mach–Zehnder interferometry [17] , [18] , [19] or spectroscopy of edge channels [20] , [21] , [22] . This situation bears strong analogies with the spin-charge separation of conventional 1D wires, except that the two spin species are carried by two separated edge channels. The direct observation of the neutral and charge eigenmodes is thus particularly favourable in the filling factor 2 case as, contrary to a conventional wire, each spin channel can be individually addressed because of their spatial separation. Still, the observation remains challenging as transport properties remain unaffected up to GHz frequencies, where the wavelength of the eigenmodes becomes comparable to the propagation length of a few microns. Many experimental works have studied charge transport in quantum Hall edge channels and interaction effects between co-propagating and counterpropagating edge channels either in time [23] , [24] , [25] , [26] or in frequency [27] , [28] , [29] , [30] domains. However, none directly addressed the separation in charge and neutral modes as the individual control of edge channels was missing. In this work, by addressing edge channels individually, we provide a direct observation of the neutral-charge eigenmodes. Using a driven mesoscopic capacitor ( Fig. 1a , see Methods for details), a sinusoidal charge density wave or edge magnetoplasmon (EMP) is induced at pulsation ω and position x =0 in channel 1, thus creating a current i 1 ( x =0, ω ) (with i 1 ( x , t )= i 1 ( x , ω ) e − iωt ). As initially introduced in the context of a non-chiral 1D wire [31] and later developed for chiral edge channels [15] at filling factor 2, Coulomb interaction during propagation can be described as the scattering of the charge density waves. For the case of filling factor 2 of interest here, scattering properties of EMPs are encoded in the 2 × 2 scattering matrix S that relates the amplitudes of the output EMP in channels 1 and 2 after propagation length l to the amplitudes of the input EMP at x =0. After an interaction length l =3.2±0.4 μm, both edge channels reach a quantum point contact (QPC), which is used to transmit or reflect channels 1 and 2. 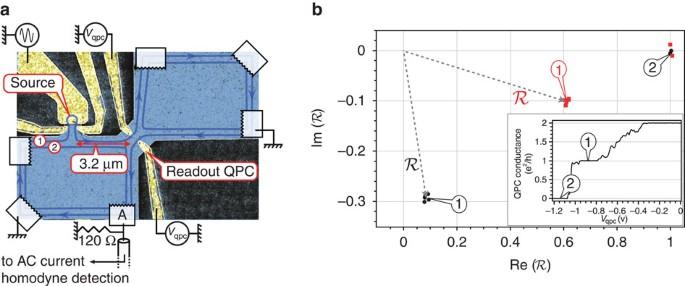Figure 1: Schematics of the sample and principle of the experiment. (a) Schematic illustration of the experiment based on the scanning electron microscopy picture of the sample. The two edge states of filling factor 2, are depicted in blue. A mesoscopic capacitor used as the source is capacitively coupled to the outer channel only, and the EMP is generated by a sine drive of variable frequency. The source is placed 3.2±0.4 μm before a QPC whose reflection can be varied so as to enable selective readout of the current in both edge states. The figure shows the setup in configuration 1 when channel 2 only is reflected. (b) RatioforMHz (black dots) and 5,500 MHz (red squares) in the complex plane. The principle of measurement is illustrated:is calculated from the ratio of the total current measured in configuration 2 and the current in the inner channel (configuration 1). The grey arrow is the complex vector representingin the complex plane. (Inset) DC measurement of the conductance of the QPC, as a function of the gate voltageVqpc, illustrating configuration 1 and 2. Figure 1b presents the principle of measurement for two typical sets of data (for f =1.3 and 5.5 GHz). In configuration 1, channel 1 is transmitted and channel 2 is reflected. The current in channel 2 resulting from the interaction, denoted i 2 ( l , ω ), can then be measured in ohmic contact A , with i 2 ( l , ω )= S 21 ( l , ω ) i 1 (0, ω ). When the QPC is closed (configuration 2), both channels are reflected so that the total collected current in A is i 1 ( l , ω )+ i 2 ( l , ω )=( S 11 ( l , ω )+ S 21 ( l , ω )) i 1 (0, ω ). Consequently, the ratio of the currents collected in these two configurations yields the complex quantity , which encodes the effect of Coulomb interaction on the propagation along the edge states. Figure 1: Schematics of the sample and principle of the experiment. ( a ) Schematic illustration of the experiment based on the scanning electron microscopy picture of the sample. The two edge states of filling factor 2, are depicted in blue. A mesoscopic capacitor used as the source is capacitively coupled to the outer channel only, and the EMP is generated by a sine drive of variable frequency . The source is placed 3.2±0.4 μm before a QPC whose reflection can be varied so as to enable selective readout of the current in both edge states. The figure shows the setup in configuration 1 when channel 2 only is reflected. ( b ) Ratio for MHz (black dots) and 5,500 MHz (red squares) in the complex plane. The principle of measurement is illustrated: is calculated from the ratio of the total current measured in configuration 2 and the current in the inner channel (configuration 1). The grey arrow is the complex vector representing in the complex plane. (Inset) DC measurement of the conductance of the QPC, as a function of the gate voltage V qpc , illustrating configuration 1 and 2. Full size image Inter-edge oscillations of EMP The experimental data for are presented in Fig. 2 (coloured dots), in the complex plane. The colour code gives an insight of the driving frequency f . Globally, we observe that draws a spiral in the complex plane. For f =0.7 GHz, we observe that , reflecting the fact that the current injected in the outer channel remains in this channel ( ). At low frequencies ( f <2 GHz), is mainly imaginary, as expected for a capacitive coupling between the two edge states. As frequency increases, winds around, reaching a maximum for GHz, meaning that 75% of the charge density wave has been transferred to the inner channel. For increasing f , continues to spiral, decreasing to , then increasing again above 9 GHz (for clarity, the corresponding data are not shown on Fig. 2 but the modulus and phase of in the range 9 GHz ≤ f ≤11 GHz are shown on Fig. 4). This behaviour demonstrates coherent oscillations of the charge density wave from one edge to the other as the driving frequency f is varied. These oscillations can be understood in a simple manner. Taking here as eigenmodes (this assumption is discussed later) the symmetric charge mode and the antisymmetric neutral mode , the current can be decomposed in the eigenbasis as , where i ρ / n are the coordinates in the eigenbasis, . 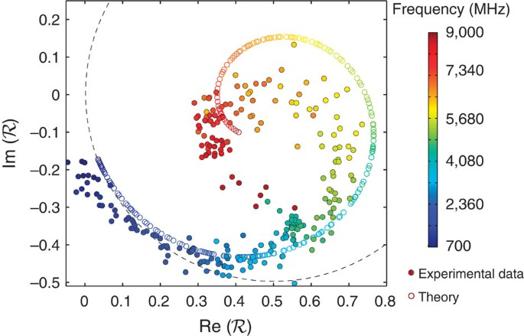Figure 2: Inter-channel oscillations. Complex ratioin the complex plane. The colour code indicates the frequencyfof the excited EMP. Experimental data (coloured dots) are compared with simulations. The grey dashes show a simulation of both short- and long-range model, without relaxation. Coloured hollow circles present a simulation of the long-range model with relaxation, for parametersps,τq=124 ps (such thatτ=81 ps) andτr=4.1 ps. Their propagation reduces to a phase factor , where v ρ / n are the phase velocities of the charge and neutral modes, respectively, with: Figure 2: Inter-channel oscillations. Complex ratio in the complex plane. The colour code indicates the frequency f of the excited EMP. Experimental data (coloured dots) are compared with simulations. The grey dashes show a simulation of both short- and long-range model, without relaxation. Coloured hollow circles present a simulation of the long-range model with relaxation, for parameters ps, τ q =124 ps (such that τ =81 ps) and τ r =4.1 ps. Full size image where we have assumed in equation (4) that the charge mode propagates much faster than the neutral mode, , such that . The term in equation (4) shows that the oscillation stems from the progressive phase shift between the charge and neutral components of the EMP propagating at different velocities. In the complex plane, should describe a circle of radius 1/2 centred at (1/2, 0), with angle when the frequency is varied. At low frequency, the propagation length l is much smaller than the wavelength of the neutral mode λ n =2 πv n / ω and propagation effects can be neglected. One then recovers the well-established [32] , [33] RC-circuit limit where starts from and for , with . can be expressed in terms of discrete elements R K and C μ , (see Methods ). C μ is the electrochemical capacitance given by the series association of a quantum capacitance for each channel (where v is the velocity in the edge channels in the absence of inter- or intra-edge channel interactions) and the geometrical capacitance between channels C . The resistor is R K = h / e 2 , the series combination of a charge-relaxation resistance R K /2 for each channel. This corresponds to the low-frequency velocity . At higher frequencies, the propagation length becomes comparable to the wavelength of the neutral mode, and propagation effects cannot be ignored. Using equation (4), the trajectory followed by in the complex plane then gives a direct access to the neutral mode velocity v n ( ω ) or, in an equivalent way, to the ω dependence of the wave vector k n ( ω ) (the dispersion relation) related to the phase velocity by . One can see on Fig. 2 that when the frequency is increased, follows the expected circle for f< 4 GHz (equation (4) is plotted in black line). However, for frequency ranging from 4 to 9 GHz, data points deviate from the expected circle and the experimental curve seems to spiral down towards a state where the charge density wave is evenly distributed between both channels with . This can be understood as a dissipation of the EMP during propagation and can be accounted for by introducing an imaginary part in the wave vector k n ( ω ). These considerations bring to light the remarkable robustness of the Nyquist diagram presented on Fig. 2 . Separation between the charge and neutral mode show up in the inter-edge oscillations revealed by the winding of around the point (1/2, 0), which corresponds to an equal repartition of the EMP. This feature, clearly visible on Fig. 2 in spite of dissipation, does not depend on the details of the interaction. The interaction characteristics are encoded in the dispersion relation k n ( ω ) or equivalently in the ω dependence of the phase Ф( ω ). To depict interactions, the most frequently used approach is a zero-range model [9] , [11] , [27] . It has no characteristic length, so that the velocity v n is frequency independent: . Because v n is frequency independent, S 21 draws a circle with a linear ω dependence of the phase Ф( ω ) ω . Any deviation from this linear dependence reflects the existence of a finite range in the interactions that can be unveiled through a careful study of the frequency dependence of . 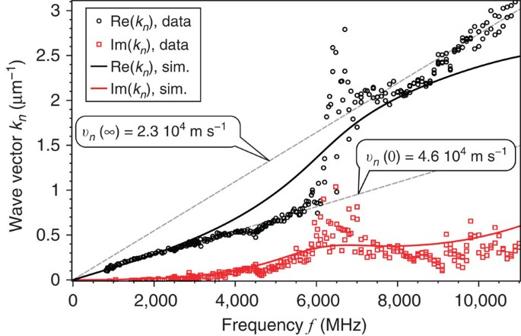Figure 3: Dissipation and dispersion of the neutral mode. Real and imaginary parts of the wave vectorkn(ω)=ω/vn(ω).exhibits two non-dispersive regimes: at low frequency (f<6 GHz),vn(0)=4.6 × 104m s−1, whereas at high frequency (f7 GHz),vn(∞)=2.3 × 104m s−1. Im(kn)≠0 indicates damping. Simulations (in black and red line) are proposed with parametersps,τq=124 ps (τ=81 ps) andτr=4.1 ps. Figure 3 presents our measurements of the dispersion relation k n ( ω ) where the complex value of k n is extracted from equation (4). As already mentioned, the existence of an imaginary part Im( k n ) in the wave vector k n signals the presence of dissipation. Two non-dispersive regimes are observed: at low frequency, , with v n (0)=4.6±0.6 × 10 4 m s −1 . This regime of constant velocity with respect to frequency is consistent with a short-range description of interactions in the low-frequency limit. However, for f >6 GHz, a second linear dispersion relation regime appears , with v n (∞)=2.3±0.3 × 10 4 m s −1 . We attribute this decrease of v n to the finite range of interactions. To go beyond this qualitative discussion, we now rely on a quantitative comparison between our experimental data for and various models of intra-edge and inter-edge interaction. Figure 3: Dissipation and dispersion of the neutral mode. Real and imaginary parts of the wave vector k n ( ω )= ω / v n ( ω ). exhibits two non-dispersive regimes: at low frequency ( f <6 GHz), v n (0)=4.6 × 10 4 m s −1 , whereas at high frequency ( f 7 GHz), v n (∞)=2.3 × 10 4 m s −1 . Im( k n )≠0 indicates damping. Simulations (in black and red line) are proposed with parameters ps, τ q =124 ps ( τ =81 ps) and τ r =4.1 ps. Full size image Comparison between model and data In Fig. 4 , experimental data for and are presented as a function of driving frequency f . At low frequency, the RC-circuit behaviour is recovered and the agreement with the experimental data is good in the range 0.7–3 GHz, with a value of ps extracted from the low-frequency regime of the dispersion relation. However, this RC-circuit model (green small dashes) does not predict oscillations. The zero-range interaction model, obtained by locally coupling the electrostatic potential of the edges to the charge densities (see Methods and Fig. 5 ) for which the velocity is frequency independent, is plotted in dashed red line. As already discussed, it does predict the oscillations, but fails to describe accurately the regime of high frequencies (3–11 GHz). Once , which prescribes the low-frequency behaviour, is fixed, no other parameter is to be fixed for the zero-range model. 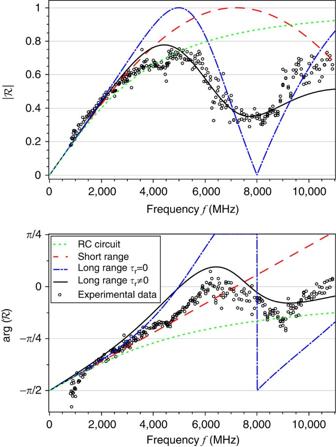Figure 4: Data-model comparison. andas a function of drive frequencyf. Experimental data (black circles) are compared with RC-circuit (green small dashes), short-range model (red dashes), long-range model without damping (blue dash-dotted line) and long-range model with relaxation (black plain line). Parameters used areps,τq=124 ps (τ=81 ps) andτr=4.1 ps. Figure 4: Data-model comparison. and as a function of drive frequency f . Experimental data (black circles) are compared with RC-circuit (green small dashes), short-range model (red dashes), long-range model without damping (blue dash-dotted line) and long-range model with relaxation (black plain line). Parameters used are ps, τ q =124 ps ( τ =81 ps) and τ r =4.1 ps. 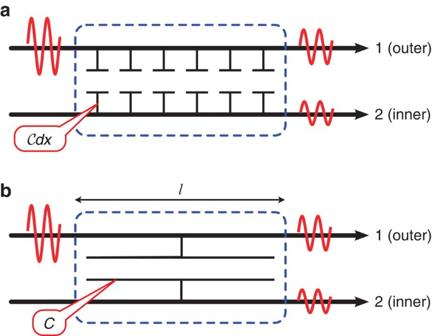Figure 5: Schematics of the zero-range and long-range interaction model. For the zero-range model (a), the charge densitiesρi(x,ω) are locally coupled to the electrostatic potentialuj(x) by the capacitance matrix per unit length,ρi(x,ω)=Cijuj(x,ω). For the long-range model (b), the potential in each edgeujis supposed to be uniform and coupled to the total chargesqiby the capacitance matrix Full size image Figure 5: Schematics of the zero-range and long-range interaction model. For the zero-range model ( a ), the charge densities ρ i ( x , ω ) are locally coupled to the electrostatic potential u j ( x ) by the capacitance matrix per unit length, ρ i ( x , ω )=C ij u j ( x , ω ). For the long-range model ( b ), the potential in each edge u j is supposed to be uniform and coupled to the total charges q i by the capacitance matrix Full size image To capture these features, an heuristic long-range model has been developed (see Methods and Fig. 5 ) based on a discrete element description [34] , [35] . An effective range on the order of the propagation length l is introduced by assuming that the electrostatic potentials of each edge state are constant over l , and by coupling these potentials to the total charges in the channels via a capacitance C . This long-range model depends on two timescales τ = R K C and τ q = R K C q = l / v such that the velocity v n ( ω ) becomes frequency dependent, (with ) and . An intrinsic dissipation inside each edge channel that accounts for the damping of the charge oscillations is introduced through the parameter γ ( ω ). We choose the following ω dependence, γ ( ω )= ω 2 τ r , which is still compatible with a discrete-circuit element description at low frequency. Dissipation modifies the value of the resistance in the RC-circuit description: a resistor of is added in series with the charge-relaxation resistor R K /2. Putting first τ r =0 (no dissipation), this long-range interaction model captures already both the low-frequency behaviour and the period of oscillation (see the blue dash-dotted curve on Fig. 4 ) from which we extract τ q =124±5 ps (which implies τ =81±4 ps because we have set ps). A good agreement with experimental data including dissipation can then be obtained using τ r =4.1±1 ps (black curve on Fig. 4 ). Note that the value of τ r extracted from our data is rather small, , such that the low-frequency regime is not strongly affected. From the evaluated value of τ q , we also deduce m s −1 , consistently with the velocity v n (∞)=2.3 × 10 4 m s −1 extracted from the dispersion relation. These values are compatible with the assumption estimating the charge velocity from experiments performed with similar samples [36] . Kumada et al . [36] indeed find a charge velocity of a few 10 6 m s −1 at filling factor 2 for an ungated 2D electron gas. Their sample characteristics are close to ours, it is made from a gallium-arsenide heterostructure, the electron gas has a density of 1.2 × 10 15 m −2 and mobility μ =2.1 × 10 6 cm 2 V −1 s −1 (close to our values, see Methods ), and the sample edges are defined by chemical etching (as ours). Simulations of the dispersion relation with the same parameters are also presented in Fig. 3 . The overall behaviour of Re( k n ) is well rendered, though not as abrupt, the change in the velocities is as expected described by the long-range interaction. In the meantime, Im( k n ) is also correctly depicted with our choice of dissipation for the EMP: γ ( ω )= ω 2 τ r . Nature of the eigenmodes Throughout the paper, the case of symmetric edge channels has been considered that naturally leads to the existence of pure charged and neutral eigenmodes. As there is no reason for both edge channels to have identical propagation properties, one should consider in full generality the decomposition , where the eigenmodes and are parametrized by the angle θ : The case θ =0 corresponds to completely independent channels, whereas θ = π /2 corresponds to the strong coupling case where the eigenmodes are the charged (+= ρ ) and neutral (−= n ) modes. As already discussed, the latter situation occurs in the case of identical edge channels but can also occur for non-identical channels as long as the inter-channel interaction is strong enough (see Methods ). Any other intermediate case corresponds to partially charged eigenmodes for which one can define the ratio r of the total charge carried by modes − and + from the expression of the eigenmodes, equation (5): . For θ = π /2, the contribution of the antisymmetric mode to the current is 0, reflecting its neutrality. In this general case, the expressions for S 21 and S 11 + S 21 , and thus for the measured quantity , differ from equations (2), (3), (4): Equation (9) shows that S 21 describes coherent oscillations from channel 1 to channel 2, whose amplitudes are given by the factor sin θ . This amplitudes only reaches unity at strong coupling θ = π /2, the only regime where a complete charge transfer from one channel to the other can be achieved. S 11 + S 21 is also affected and oscillates (either with frequency f or length l ), reflecting the fact that in this general case, the charge mode is no longer an eigenmode such that the total current i 1 + i 2 oscillates instead of simply accumulating a phase. As a result, still follows a circle in the complex plane but with a θ -dependent radius and centre. From these general expressions and the comparison with our experimental data, one can assess that the eigenmodes are indeed the charge and neutral ones, within an accuracy of r =0±0.1 for the charge ratio between the eigenmodes. The first argument comes from the low-frequency behaviour of where dissipation can be safely neglected. Both the modulus and the phase follow a linear ω dependence but with two different θ -dependent slopes, , . By measuring the ratio of these slopes, one can directly measure the angle θ . Remarkably, in the strong coupling case, , data points for and should follow the exact same frequency dependence in the low-frequency regime. Data points in the low frequency 0.9–4.5 GHz range are plotted on Fig. 6 , with their linear fits. A linear fit for (in the 0.9–2 GHz range, as approaches its maximum for GHz) is presented in black plain line, yielding . Similarly, is fitted in red line in the range 1.2–4.5 GHz range, with . Data below 1.2 GHz are not used in the fitting procedure because of their dispersion, as, at low frequency, is obtained from the ratio between two small currents. The slope of , that is, the value of for small ω , is determined with a 10% accuracy. It thus defines two bounds (dashed blue lines) that correspond to the slopes of for θ =90+11° (upper bound) θ =90−11° (lower bound). These extremum values of the angle θ correspond to a charge ratio =±0.1. Our data points for fall between these bounds that assesses the neutrality of the slow mode with a 10% accuracy. The second argument comes from the study of the full trajectory of in the complex plane. From the amplitude of the oscillations of the EMP from one edge to the other, a lower bound for θ can be obtained, θ ≥74° corresponding to . This lower bound is obtained by assuming that the amplitude of the oscillation is only limited by the value of θ and neglects fully the dissipation. Taking into account dissipation, the full trajectory and in particular the position of the centre of the spiral described by confirm θ =90° with the same accuracy of ±11° as in the low-frequency regime. 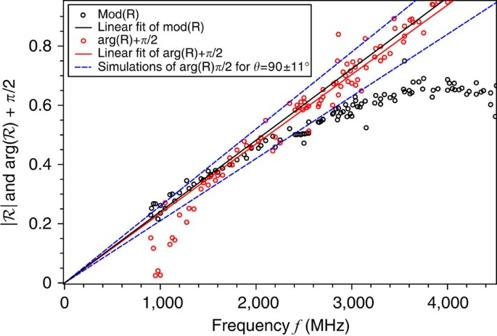Figure 6: Test of the nature of eigenmodes. In the low-frequency regime,andare presented in black and red circles, respectively, and fitted with linear functions (black and red lines). The slope ofis obtained with a 10% accuracy, defining two bounds drawn in blue dashes associated toforand. Data points fall between these bounds confirming. Figure 6: Test of the nature of eigenmodes. In the low-frequency regime, and are presented in black and red circles, respectively, and fitted with linear functions (black and red lines). The slope of is obtained with a 10% accuracy, defining two bounds drawn in blue dashes associated to for and . Data points fall between these bounds confirming . Full size image We have directly observed the collective excitations of two coupled chiral edge channels at filling factor 2 and demonstrated that it consisted in an antisymmetric neutral mode and a symmetric mode carrying the charge. By creating selectively a charge density wave at frequency f in the outer edge and measuring the current transferred to the inner one, we have observed oscillations as a function of frequency that reflect the phase shift between the charge and neutral modes. The minima of these oscillations correspond to integer values of the ratio l / λ n between the propagation length and the wavelength of the neutral mode. From these measurements, we have deduced the dissipation and dispersion relation of the neutral mode, k n ( ω ). We have observed two non-dispersive regimes, corresponding to a phase velocity v n =4.6±0.6 × 10 4 m s −1 at low frequency and v n (∞)=2.3±0.3 × 10 4 m s −1 at high frequency. Comparing our results with various models of inter-edge interactions, our results show that edge channel propagation differs from the ideal Luttinger limit of dissipationless propagation with short-range interaction, but rather agrees with a model of dissipative channels coupled through a long-range interaction. Dissipation could be caused by the internal structure of compressible edges, leading to a coupling of EMP to acoustic modes [37] , [38] , but a non-ambiguous diagnosis will require further investigation. Sample description The sample is realized in a standard GaAs/Ga(Al)As 2D electron gas located 100 nm below the surface, of density n =1.8 × 10 15 m −2 and mobility μ =2.4 × 10 6 cm 2 V −1 s −1 . The sample is then patterned using e-beam lithography and chemical etching of the heterojunction, and by deposition of metallic gates at the surface. The electron gas is contacted using Gold/Germanium ohmic contacts schematically represented as white squares on Fig. 1a . The sample is placed in a strong magnetic field B =3.65 T so as to reach filling factor 2 in the bulk (see Fig. 1a ). A driven mesoscopic capacitor (described in Büttiker et al . [39] and Parmentier et al . [40] ) is used to selectively inject current in the outer-edge channel (labelled 1). The mesoscopic capacitor comprises a small portion of the electron gas (of submicronic size), called a quantum dot, capacitively coupled to a metallic top gate, see Fig. 1a . A QPC is used to fully transmit the outer-edge channel (1) inside the dot, whereas the inner channel (2) is fully reflected. A sine drive of frequency is applied on the metallic top gate deposited on top of the dot, so that an EMP of frequency f is capacitively induced in the outer channel, carrying a current i 1 (0, ω ). The propagation takes place on a length μm, during which channels are interacting. The EMP then reaches a QPC, which allows to reflect or transmit selectively each edge channel. The reflected AC current flows towards ohmic contact A, situated at distance μm from the QPC, and where the total current is measured. Note that the propagation after the QPC, on length L , is irrelevant in the analysis of the data: according to equation (2), measuring the total reflected current in ohmic contact A is equivalent, up to a phase factor , to measuring the total current flowing right after the QPC. The current is measured using a wideband room-temperature homodyne detection. A set of microwave filters and room-temperature low-noise amplifiers enables a proper measurement in the 0.7–11 GHz range. Note that does not depend on the total gain of the amplifying detection scheme, which varies considerably in the studied frequency range. Each reported data point results from a simple averaging protocol, and the statistical analysis is in good agreement with the observed dispersion of the experimental data. At low frequency (<1 GHz), the quality of our measurements is limited by the bandwidth of our filters and amplifiers. At high frequency (>10 GHz), it is limited for the same reason, combined with increased attenuation of the output RF coaxial cables. Experiments were performed in a dilution fridge of base temperature 50 mK. By performing Coulomb thermometry on the mesoscopic capacitor [32] , we have calibrated the electronic temperature to T el =100±10 mK. Elements of theory In the integer quantum Hall regime, edge magnetoplasmons in channel 1 (outer) and 2 (inner) are described by a chiral bosonic field ( i =1, 2). In this approach, the two edge channels are bosonized in the spirit of Wen’s description of quantum Hall edges as chiral Luttinger liquids [41] . The current in channel i is then determined by , whereas the charge density is . Both are related via the current conservation equation. In Fourier space, the motion of the chiral field along the edge obeys: where v i is the velocity of edge channel i in the absence of interactions and u i the potential in edge channel i . The term γ ( ω ) models an intrinsic dissipation inside the edge states that accounts for the damping of the charge oscillations. Equation (13) can be rewritten as a function of the current in edge channel i : First, let us consider the non-damped case γ ( ω )=0. The short-range description of the interaction can be obtained by coupling locally the charge densities ρ i ( x , ω ) to the local electrostatic potential u i ( x , ω ) via distributed capacitances C ij (see Fig 5 ): ρ i ( x , ω )= C ij u i ( x , ω ), where C =− C 21 =− C 12 accounts for the coupling between channels, whereas C ii describes intra-channel interactions in edge channel i . These coupled equations are solved when working in the eigenbasis that diagonalizes the velocity matrix, . In the absence of inter-channel interaction, , the channels are not coupled ( ), but the velocities are renormalized by intra-channel interactions: . In the presence of inter-channel interactions ( ), new eigenmodes denoted by + and − and defined by equations (5)–(8), with θ ≠0 appear. The velocities and coupling angle θ are expressed as functions of the velocity matrix elements by: As a consequence of the zero range of the interaction, the velocities are ω independent. Note that the domain θ [0, π /2] corresponds to the expected situation where, in the absence of inter-channel interaction, the outer-edge channel velocity is greater than the inner one, . The scattering matrix describing the coupled propagation can then be straightforwardly calculated, yielding equations (9)–(11). The charge (+ → ρ ) and neutral (− → n ) eigenmodes are recovered for θ = π /2, which always occurs for identical edge channels, , but also for strong enough inter-channel interaction, . As demonstrated above, this limit corresponds to the experimental situation. In this case, the velocity becomes , with and . The case corresponds to total influence between edge channels, , and such that . At low enough frequency, this short-range model should describe correctly the coupling between channels. As discussed in the paper, this corresponds to the RC-circuit description, , where C = l C is the total geometrical capacitance and C q = le 2 /( hv ) the total quantum capacitance. At higher frequencies, a way to account for long-range interaction is to assume that the potentials u i are uniform in the whole-edge channel i , and related to the total charges in the 1D wires: q i = C ij u j with C = C 21 = C 12 (see Fig. 5 ). In this description, the effective interaction range is given by the co-propagating length l itself. The same calculations can be performed to calculate S 21 and in full generality (even for γ ( ω )≠0 as detailed below). From now on, we assume that θ = π /2 as demonstrated in this article. Taking into account the damping in this model ( γ ( ω )≠0), we now obtain: For γ ( ω )=0, S 21 also draws a circle of radius 1/2 centred on (1/2, 0) in the complex plane, but in contrast to the short-range case, the ω dependence of the phase deviates from the linear law θ ( ω ) ω , which shows that the velocity v n ( ω ) becomes frequency dependent. This frequency dependence is related to the two timescales τ and τ q introduced by the model. At low frequencies, one recovers the RC-circuit description with . For γ ≠0 and choosing γ ( ω )= ω 2 τ r , as mentioned above, the RC-circuit description is modified: a resistor of is added in series with the charge-relaxation resistor R K /2. How to cite this article: Bocquillon E. et al . Separation of neutral and charge modes in one-dimensional chiral edge channels. Nat. Commun. 4:1839 doi: 10.1038/ncomms2788 (2013).